Reply to: Available data do not rule out Ctenophora as the sister group to all other Metazoa 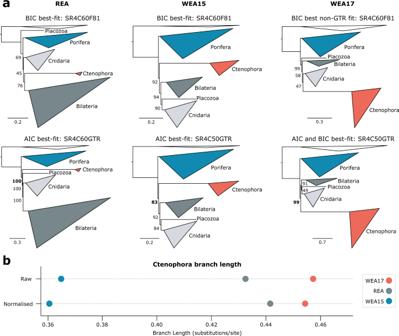Fig. 1: Unpartitioned recoding reanalyses and ancestral ctenophore branch lengths. aReanalyses of SR4 recoded animal phylogeny datasets REA, WEA15, and WEA17 without using partitioning. Consensus trees from reanalyses with best-fitting F81-based models are shown in the top row and those from reanalyses with best-fitting GTR-based models are shown in the second row. Model-fitting results reported above each tree compared both F81 and GTR-based models (including site-homogeneous F81 and GTR). Ultrafast bootstrap support for Porifera-sister is shown in bold for the GTR-based analyses. Models are as specified in R&M1.bLength in substitutions/site of the ancestral branch of the Ctenophore clade for each dataset as analysed at the amino acid level using standard partitioned phylogenomics with site-homogeneous models (i.e., analysis level ‘L1’ of R&M1). ‘Raw’: branch length extracted directly from the resultant tree, ‘Normalised’: branch length divided by total tree length (and then multiplied by the mean total tree length of the three datasets for presentation in comparison to Raw). Unpartitioned, site-heterogeneous, SR4-recoded animal phylogenomics SR4 [21] recoded phylogenomic analyses were performed on the REA, WEA15, and WEA17 datasets from R&M [1] using IQ-tree version 1.6.12 [20] and employing 1000 ultrafast bootstrap replicates [22] . All analyses performed here were unpartitioned in order to test whether poor resolution and inconsistent results between datasets are ascribable to (i) SR4 recoding (as contended by W&H [2] ) or (ii) simple, flat F81 exchangeabilities (as proposed here and in R&M), which were always better-fitting than GTR exchangeabilities when combining partitioning, recoding and site-heterogeneous models in R&M [1] . The logic behind this is that when a single model is applied to the entire phylogenomic dataset rather than separate models to each partition, then there may be enough data for site-heterogeneous models with GTR, rather than simpler F81, exchangeabilities to fit best when recoding is applied. ModelFinder [23] in IQ-tree was used to assess the best-fitting models under both the AIC and BIC. The site-homogeneous models F81 and GTR were tested, as well as pairings of each of these exchangeability matrices with SR4 recoded derivations (from R&M [1] ) of the site-heterogenous C10, C20, C30, C40, C50, and C60 precomputed CAT models [19] . All site-heterogeneous models also incorporated 4 discrete gamma categories to help accommodate rate heterogeneity across sites. For example, the model ‘SR4C60GTR’ (see naming as applied in Fig. 1a ), is SR4 recoded, employs GTR exchangeabilities, the 60 site frequency categories from C60, and 4 discrete gamma categories for rate heterogeneity. Each dataset was analysed under the best fitting GTR-based model (GTR-based models always fit best under AIC), as well as under the best-fitting F81-based model (best-fitting under BIC for REA and WEA15), enabling comparison of the resultant maximum likelihood consensus trees and support values between GTR-based and F81-based analyses, as well as with previous F81-based partitioned analyses performed in R&M [1] . Ancestral Ctenophora branch length as an LBA severity measure The long ancestral ctenophore branch (i.e., the internal branch leading to the extant ctenophores in the animal tree of life) has been suggested to cause LBA between Ctenophora and non-animal outgroups, producing tree topologies supporting Ctenophora as sister to all other animals [1] , [7] , [8] , [10] , [12] . We contend that the longer this branch is (i.e., the more substitutions per site along this branch) in a given dataset (branch length may vary due to substitution model applied, differing gene and site content, variation in alignment and orthology errors, etc.) the more difficult it will be to overcome potential LBA of Ctenophora towards the root of the animal tree when analysing that dataset. We extracted this branch length value from the maximum likelihood consensus trees resulting from standard partitioned phylogenomics of the REA, WEA15, and WEA17 datasets performed in R&M (i.e., named analysis level ‘L1’ in R&M [1] ). Branch lengths were plotted in Fig. 1b for comparison across datasets, both in ‘Raw’ form (as directly extracted from the consensus trees) and in ‘Normalised’ form (raw branch length divided by total tree length for that dataset, then multiplied by the average total tree length of the three datasets). Reporting summary Further information on research design is available in the Nature Portfolio Reporting Summary linked to this article.